Non-enzymatic chemistry enables 2-hydroxyglutarate-mediated activation of 2-oxoglutarate oxygenases Accumulation of ( R )-2-hydroxyglutarate in cells results from mutations to isocitrate dehydrogenase that correlate with cancer. A recent study reports that ( R )-, but not ( S )-2-hydroxyglutarate, acts as a co-substrate for the hypoxia-inducible factor prolyl hydroxylases via enzyme-catalysed oxidation to 2-oxoglutarate. Here we investigate the mechanism of 2-hydroxyglutarate-enabled activation of 2-oxoglutarate oxygenases, including prolyl hydroxylase domain 2, the most important human prolyl hydroxylase isoform. We observe that 2-hydroxyglutarate-enabled catalysis by prolyl hydroxylase domain 2 is not enantiomer-specific and is stimulated by ferrous/ferric ion and reducing agents including L -ascorbate. The results reveal that 2-hydroxyglutarate is oxidized to 2-oxoglutarate non-enzymatically, likely via iron-mediated Fenton-chemistry, at levels supporting in vitro catalysis by 2-oxoglutarate oxygenases. Succinic semialdehyde and succinate are also identified as products of 2-hydroxyglutarate oxidation. Overall, the results rationalize the reported effects of 2-hydroxyglutarate on catalysis by prolyl hydroxylases in vitro and suggest that non-enzymatic 2-hydroxyglutarate oxidation may be of biological interest. Mutations to genes encoding for enzymes of the tricarboxylic acid (TCA) cycle, including isocitrate dehydrogenase (IDH1/2), can lead to substantial increases in cellular metabolites, as observed in both genetic diseases (germline mutations) [1] and in cancer (somatic mutations) [2] . Elevated levels of ( R )-2-hydroxyglutarate (( R )-2HG) produced by a ‘gain-of-function’ mutation to IDH1/2 result in massively increased concentrations of ( R )-2HG (up to 10 mM) and decreases in 2-oxoglutarate (2OG) levels [3] . It is proposed that elevated levels of succinate, fumarate and ( R )-2HG in humans cause pro-oncogenic effects via inhibition of Fe(II)/2OG dependent oxygenases [4] , [5] , [6] . 2OG oxygenases are involved in chromatin regulation by modification of both nucleic acids, for example 5-methylcytosine oxidation, and histone tails via N ε -methyl lysine residue demethylation [7] . 2OG oxygenases also play pivotal roles in the cellular and physiological responses to hypoxia by regulation of the levels and activity of the hypoxia-inducible transcription factor (HIF), which is an α,β-heterodimeric protein that activates transcription of an array of genes under conditions of low oxygen availability [8] . The prolyl hydroxylase domain enzymes (PHDs, EGLN 1-3) catalyse hydroxylation of prolyl-residues in HIF-α isoforms, a post-translational modification that signals for the proteosomal degradation of HIF-α [9] . Factor inhibiting HIF (FIH) catalyses hydroxylation of an asparaginyl-residue resulting in reduction of HIF-α mediated transcription by reducing binding of HIF to transcriptional co-activators [9] . HIF upregulation activates the transcription of a gene array, which is proposed to promote tumour growth via increased angiogenesis. It is therefore proposed that inhibition of HIF hydroxylases by TCA cycle metabolites and ( R )-2HG may be linked to tumour development [10] . It has been reported that elevated ( R )-2HG levels caused by IDH mutations may indeed inhibit PHD action in cells resulting in HIF-activated transcription [11] , though our work and that of others has indicated that ( R )- and ( S )-2HG are only weak inhibitors for the HIF hydroxylases [12] , [13] , [14] . It is also possible that elevated ( R )-2HG concentrations inhibit chromatin-modifying 2OG oxygenases [15] , [16] . Although it has been widely perceived that HIF is an oncoprotein, HIF-α isoforms can act as tumour suppressors in certain tumours [17] , [18] , [19] , [20] . Thus, PHD inhibition may be of therapeutic interest for such cancers. In contrast to the paradigm that TCA cycle metabolite and ( R )-2HG-mediated inhibition of 2OG dependent oxygenases is pathogenic, it has been recently reported that ( R )-, but not ( S )-2HG, actually stimulates PHD activity, both with isolated components and in cells, so reducing HIF levels, leading to enhanced proliferation of astrocytes [21] . However, the effect of ( R )-2HG on PHD2 activity and its potential relation to cancer remain controversial [11] , [13] , [15] , [21] . The consensus catalytic mechanism for 2OG dependent oxygenases proceeds via formation of an enzyme–Fe(II)–2OG–substrate complex that binds dioxygen; subsequent oxidative decarboxylation of 2OG yields succinate and carbon dioxide and a reactive Fe(IV)–oxo intermediate, which performs the two-electron substrate oxidation ( Fig. 1 , refs 22 , 23 ). Koivunen et al. [21] have proposed that 2OG can be formed enzymatically in the PHD2 active site as a product of ( R )-2HG, but not ( S )-2HG, oxidation, and suggested that this occurs via an Fe(III)–superoxide intermediate. While prime substrate C-H cleavage by such intermediates has precedent in some non-haem iron oxygenases [24] , C-H cleavage in a co-substrate is unprecedented in 2OG oxygenase catalysis and in earlier work we did not observe that 2HG can substitute for 2OG under our standard assay conditions [14] . 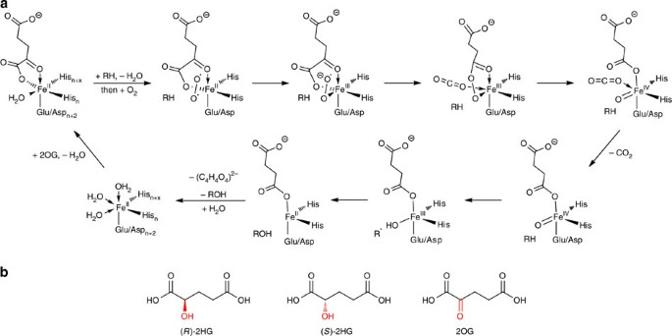Figure 1: The proposed catalytic mechanism for 2OG-dependent oxygenases. (a) Binding of dioxygen, which occurs subsequently to enzyme–substrate complex formation, results in the oxidative decarboxylation of 2OG and generation of an Fe(IV)-oxo species that enables hydroxylation. (b) Structures of 2HG (2-hydroxyglutarate) and 2OG (2-oxoglutarate). Figure 1: The proposed catalytic mechanism for 2OG-dependent oxygenases. ( a ) Binding of dioxygen, which occurs subsequently to enzyme–substrate complex formation, results in the oxidative decarboxylation of 2OG and generation of an Fe(IV)-oxo species that enables hydroxylation. ( b ) Structures of 2HG (2-hydroxyglutarate) and 2OG (2-oxoglutarate). Full size image Here we report investigations on the mechanism of the apparent activation of PHDs by ( R )-2HG and the origin of the 2HG conversion to 2OG. We show that conversion of 2HG to 2OG occurs non-enzymatically in a manner enabled by biologically relevant reducing agents including L -ascorbate and the reduced form of L -glutathione. The level of 2OG is sufficient to support catalysis by PHD2, and at least one other human 2OG oxygenase. Studies on the mechanisms of 2HG-promoted PHD2 catalysis To investigate the mechanism by which PHD activity is enabled by the presence of 2HG, MALDI-TOF-MS (matrix assisted laser desorption ionization-time of flight-mass spectrometry) based assays were performed using a peptide fragment of the HIF-1α C -terminal oxygen-dependent degradation domain (HIF-1α 556–574 , hereafter CODD) and recombinant PHD2 181–426 (hereafter PHD2). In contrast to Koivunen et al. [21] , when substituting 300 μM 2OG for 5 mM 2HG in our standard steady-state assay conditions (4 μM PHD2, 200 μM CODD; Supplementary Table 1 ), we did not observe any CODD hydroxylation after short incubation times (up to 2 h, limit of detection: ~3% CODD hydroxylation). CODD hydroxylation was observed, however, with longer incubation times (20 h) ( Fig. 2c,d ) in the presence of both ( R )- and ( S )-2HG. 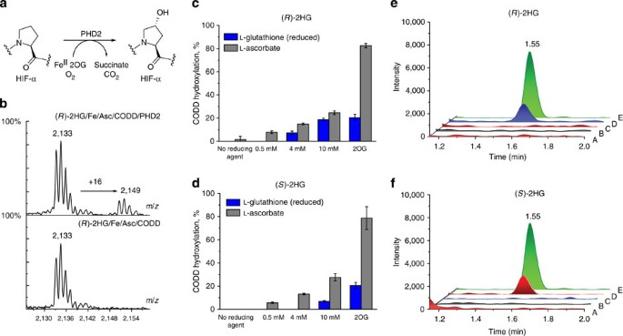Figure 2: PHD2/2HG catalysis is enabled by reducing agents. Samples containing 4 μM PHD2 (prolyl hydroxylase domain 2), 200 μMC-terminal oxygen dependent degradation domain (CODD) peptide, 5 mM (R)- or (S)-2HG, 50 μM Fe(II), 0/0.5/4/10 mML-ascorbate in Hepes 50 mM pH 7.5 were incubated for 20 h (37 °C) and then analysed by MALDI-TOF-MS or subjected to amino acid analysis. Error bars represent s.d. of the mean of triplicate assays. 2OG (2-oxoglutarate) control incubations contained 300 μM 2OG instead of 2HG. (a) The PHD2-catalysed reaction. (b) Typical MALDI-TOF-MS spectra of CODD-OH (upper) and CODD (lower). (c) Dependence of PHD2/(R)-2HG-catalysed CODD hydroxylation onL-ascorbate and GSH (glutathione). (d) Dependence of PHD2/(S)-2HG-catalysed CODD hydroxylation reaction onL-ascorbate and GSH. (e,f) Amino acid analysis results (A: 2HG, Fe(II),L-ascorbate; B: CODD, 2HG, Fe(II),L-ascorbate; C: PHD2, 2HG, Fe(II),L-ascorbate; D: PHD2, CODD, 2HG, Fe(II),L-ascorbate; E: standard containingtrans-4-hydroxyproline amino acid). Figure 2: PHD2/2HG catalysis is enabled by reducing agents. Samples containing 4 μM PHD2 (prolyl hydroxylase domain 2), 200 μM C -terminal oxygen dependent degradation domain (CODD) peptide, 5 mM ( R )- or ( S )-2HG, 50 μM Fe(II), 0/0.5/4/10 mM L -ascorbate in Hepes 50 mM pH 7.5 were incubated for 20 h (37 °C) and then analysed by MALDI-TOF-MS or subjected to amino acid analysis. Error bars represent s.d. of the mean of triplicate assays. 2OG (2-oxoglutarate) control incubations contained 300 μM 2OG instead of 2HG. ( a ) The PHD2-catalysed reaction. ( b ) Typical MALDI-TOF-MS spectra of CODD-OH (upper) and CODD (lower). ( c ) Dependence of PHD2/( R )-2HG-catalysed CODD hydroxylation on L -ascorbate and GSH (glutathione). ( d ) Dependence of PHD2/( S )-2HG-catalysed CODD hydroxylation reaction on L -ascorbate and GSH. ( e , f ) Amino acid analysis results (A: 2HG, Fe(II), L -ascorbate; B: CODD, 2HG, Fe(II), L -ascorbate; C: PHD2, 2HG, Fe(II), L -ascorbate; D: PHD2, CODD, 2HG, Fe(II), L -ascorbate; E: standard containing trans -4-hydroxyproline amino acid). Full size image 2OG oxygenase catalysis is often stimulated in vitro by L -ascorbate or other reducing agents [25] , [26] , [27] . L -ascorbate is required for PHD2 activity [14] , [25] , [28] , and is a standard component in PHD2 reaction incubations [21] , [29] ( Supplementary Table 1 ). We found that, under the steady-state conditions described above, the extent of PHD2/2HG-mediated CODD hydroxylation was dependent on L -ascorbate concentration; 20% CODD hydroxylation was observed in the presence of 10 mM L -ascorbate ( Fig. 2c,d ), ~4–7% CODD hydroxylation was observed in the presence of lower, possibly more physiologically relevant levels of L -ascorbate (0.1–0.3 mM, Supplementary Fig. 1a,b ) [30] . L -Glutathione (thiol form, GSH) is a biologically important antioxidant that plays a role in cellular protection against oxidative stress [31] . We found that GSH was also able to promote PHD2/2HG-mediated CODD hydroxylation, albeit at higher concentrations than L -ascorbate ( Fig. 2c,d ). This observation is consistent with the reduced ability of GSH to stimulate 2OG-enabled PHD2 catalysis in vitro [28] . To confirm 2HG-mediated prolyl-hydroxylation of CODD, amino acid analyses were performed; trans -4-hydroxylated proline was detected in hydrolysed PHD2/CODD assay mixtures where the assay was conducted in the presence of either ( R )- or ( S )-2HG ( Fig. 2e,f ). To test whether CODD hydroxylation was a product of catalysis, rather than a result of non specific oxidation by reactive oxidizing species (ROS) ‘leaking’ from the enzyme active site, the Fe(II)/2HG/ L -ascorbate/CODD assay mixture was incubated with 0–100 μM H 2 O 2 instead of PHD2. A +16 Da mass shift in the CODD MALDI-TOF-MS spectra was not observed under these conditions. Studies on the binding of 2HG to PHD2 We were intrigued by the differences in our results when compared with those of Koivunen et al. [21] , including the incubation time required for CODD hydroxylation to be observed, the apparent dependence on the presence of reducing agent, and our observation that in the presence of L -ascorbate no significant difference in the extent of CODD hydroxylation was seen when using ( S )- or ( R )-2HG ( Fig. 2c,d ). We therefore carried out investigations to understand the nature of the 2HG/PHD2-mediated CODD hydroxylation, including the possibility of ( R )-2HG oxidation being catalysed by PHD2, as proposed [21] . To investigate whether ( R )- and ( S )-2HG bind to the catalytic domain of PHD2, biophysical techniques were employed. First, we employed an NMR assay that measures displacement of 2OG from the PHD2–Zn(II)–2OG complex (Zn(II) is a catalytically inactive substitute for Fe(II)) [32] . Previous studies indicated very strong binding of 2OG to PHD2 ( K d =1 μM), which was not dependent on the presence of the prime substrate [33] . The NMR results showed that both ( R )- and ( S )-2HG exhibit very weak binding to PHD2 (determined K d >1 mM and >0.6 mM respectively, Supplementary Fig. 2 ). Next, we used UV–vis spectroscopy to probe for the formation of a metal-to-ligand charge transfer feature: the anaerobic PHD2–Fe(II)–2OG complex absorbs at 530 nm [25] ; however, addition of ( R )- or ( S )-2HG to PHD2–Fe(II) under anaerobic conditions did not result in the formation of any observable metal-to-ligand charge transfer feature ( Supplementary Fig. 3 ). This suggests either the absence of 2HG binding within limits of detection, or significant differences in the interaction of 2HG with the active site metal compared with 2OG. We then conducted non-denaturing MS experiments to look for stable complex formation in the presence and absence of CODD prime substrate ( Supplementary Fig. 4 ) [34] . ( R )-2HG was not observed to bind to PHD2–Fe(II) by non-denaturing MS (in contrast with 2OG), either in the absence or presence of CODD, nor was there evidence for CODD hydroxylation on analysis of PHD2–Fe(II)–( R )-2HG–CODD as there was in the presence of 2OG. Overall, we were unable to find any evidence for efficient 2HG binding to PHD2. We next considered the possibility of 2OG contamination of commercial batches of ( R )- and ( S )-2HG as a source of 2OG to elicit CODD hydroxylation. NMR and liquid chromatography-mass spectrometry (LC-MS) analyses revealed up to 0.02% (by molarity) 2OG in almost all batches (three out of four) of commercially purchased ( R )-2HG, but not ( S )-2HG (4 batches), which is equivalent to 1 μM 2OG in 5 mM ( R )-2HG (as used in standard assay conditions) ( Supplementary Fig. 5 ). 1 μM 2OG and 5 mM ( R )-2HG support similar degrees of CODD hydroxylation, detectable under single turnover conditions ( Supplementary Fig. 1c ). We further subjected ( R )-2HG to high-pressure liquid chromatography (HPLC) to remove 2OG contamination, then re-determined the IC 50 values of both ( R )- and ( S )-2HG ( Supplementary Fig. 6 ); consistent with our previous work [14] , we found that ( R )- and ( S )-2HG are both very weak inhibitors of PHD2 (IC 50 values are 23 mM and 6 mM for ( R )- and ( S )-2HG, respectively). Thus, the low levels of CODD hydroxylation observed in the absence of L -ascorbate ( Fig. 2c,d ) may reflect the presence of contaminating 2OG in commercial ( R )-2HG samples, and may also reflect differences in ( R )- and ( S )-2HG inhibition activities. Reducing agent and iron promote non-enzymatic 2HG oxidation Given the apparent ability of reducing agents to promote 2HG-mediated CODD hydroxylation ( Fig. 2c,d ), we used an antibody based assay, which gives a CODD-OH specific fluorescent signal [35] , to investigate the conditions required for CODD hydroxylation and to verify the sensitivity of our MS-based assay. Interestingly, we found that when PHD2/CODD were added after a 20 h preincubation of a mixture of ( R )- or ( S )-2HG, Fe(II) and L -ascorbate, a fluorescence signal was observed (indicative of CODD hydroxylation) after just 10 min of enzymatic activity. Fluorescence was greater in the samples containing L -ascorbate, and there was no difference between the two 2HG enantiomers ( Supplementary Fig. 7 ). This result suggested that during the course of the preincubation 2HG was oxidized non-enzymatically to 2OG, to a level sufficient to support PHD catalysis. We therefore considered it possible that the mechanism of PHD2/2HG-mediated CODD hydroxylation was via non-enzymatic 2HG oxidation to 2OG followed by PHD2/2OG mediated CODD hydroxylation. As reducing agents promote 2HG-mediated CODD hydroxylation ( Fig. 2c,d ), we investigated whether they are necessary for non-enzymatic conversion of 2HG to 2OG. Mixtures of ( R )- or ( S )-2HG with Fe(II) and different concentrations of L -ascorbate/GSH were incubated for 20 h (37 °C). 2OG formation was detected by LC-MS, and was observed in the samples containing L -ascorbate and GSH, without discrimination between ( R )- or ( S )-2HG ( Fig. 3 ). Substituting with oxidized forms of L -ascorbate and glutathione (dehydroascorbate and GSSG) resulted in little or no 2OG formation (limited 2OG formation observed in the presence of dehydroascorbate could be due to its partial reduction to L -ascorbate under the assay conditions) ( Fig. 3c,d ). Reducing agents can therefore promote the non-enzymatic oxidation of 2HG to 2OG. 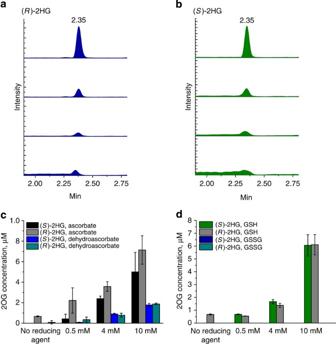Figure 3: 2HG conversion to 2OG is non-enzymatic. (a,b) LC-MS chromatograms showing 2OG formation under non-enzymatic conditions in the presence of GSH (glutathione). (c,d) Amounts of 2OG formed with different reducing agents. Error bars represent s.d. of the mean of triplicate assays. The reaction mixture was incubated for 20 h (37 °C) and contained 5 mM (R)- or (S)-2HG, 50 μM Fe(II), reducing agent (from bottom to top in (a,b): no reducing agent; 0.5 mM; 4 mM; 10 mM reducing agent). All panels in one stack in (a,b) have the same range of ion intensity (0–6.5·105). Figure 3: 2HG conversion to 2OG is non-enzymatic. ( a , b ) LC-MS chromatograms showing 2OG formation under non-enzymatic conditions in the presence of GSH (glutathione). ( c , d ) Amounts of 2OG formed with different reducing agents. Error bars represent s.d. of the mean of triplicate assays. The reaction mixture was incubated for 20 h (37 °C) and contained 5 mM ( R )- or ( S )-2HG, 50 μM Fe(II), reducing agent (from bottom to top in ( a , b ): no reducing agent; 0.5 mM; 4 mM; 10 mM reducing agent). All panels in one stack in ( a , b ) have the same range of ion intensity (0–6.5·10 5 ). Full size image We investigated the Fe(II)-dependence of non-enzymatic conversion of 2HG to 2OG and found that ascorbate- and glutathione-mediated 2HG oxidation requires the presence of either Fe(II) or Fe(III) ( Supplementary Figs 8 and 9 ). The level of 2OG produced (detected by LC-MS) was dependent on the concentration of iron. We also investigated whether other transition metals could substitute for Fe(II)/Fe(III) in this reaction, and found that metals such as Zn(II), Mn(II), Co(II), Ni(II) and Cu(II) did not promote 2OG formation. NMR studies were performed to confirm that non-enzymatic oxidation of 2HG to 2OG is Fe(II)/(III)- and reducing agent-dependent ( Supplementary Fig. 9 ). Consistent with the LC-MS results, the non-enzymatic conversion of 2HG to 2OG was observed, which was promoted by the presence of both L -ascorbate and Fe(II) ( Fig. 4a ). The time course of the reaction was investigated by NMR and showed a linear increase in 2OG generation over 20 h ( Fig. 4b ). Although, an excess of L -ascorbate/GSH relative to iron was found to be required to effectively enable the non-enzymatic reaction ( Fig. 3c,d ), physiologically relevant levels of these reducing agents [30] , [36] are able to promote 2OG formation to levels that sustain CODD hydroxylation ( Fig. 2c,d ). Notably, low amounts of 2OG were also observed after incubation of 2HG and 10 mM L -ascorbate when no Fe(II) was added ( Fig. 4a ), which could be due to trace Fe(II) contamination present in reaction components including ascorbate and H 2 O, as revealed by inductively coupled plasma-mass spectrometry (ICP-MS) analyses (at least ~1 μM Fe(II)/Fe(III), Supplementary Table 2 ). 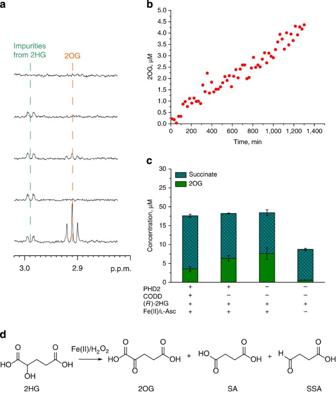Figure 4: Non-enzymatic conversion of (S)- and (R)-2HG to 2OG. (a)1H NMR spectra showing conversion of (S)-2HG (2-hydroxyglutarate) to 2OG (2-oxoglutarate). The1H spectra show the 2OG CH2COCO2H resonance. Conditions (from top to bottom): 50 μM Fe(II) and 10 mML-ascorbate; 5 mM (S)-2HG and 50 μM Fe(II); 5 mM (S)-2HG and 10 mML-ascorbate; 5 mM (S)-2HG; 5 mM (S)-2HG, 50 μM Fe(II) and 10 mML-ascorbate. Reaction mixtures were incubated for 20 h at 25 °C. All solutions were buffered with 50 mM Tris-d11(pH 7.5) and 0.02% NaN3in 90% H2O and 10% D2O. (b) Time course of non-enzymatic 2OG production as analysed by1H NMR. Conditions: 5 mM (S)-2HG, 5 μM Fe(II), 2 mML-ascorbate. (c) Succinate and 2OG production (total concentration) in the assay mixtures containing (R)-2HG. Conditions: 5 mM (R)-2HG, 5 μM Fe(II), 2 mML-ascorbate, 4 μM PHD2 (prolyl hydroxylase domain 2), 128 μM CODD (C-terminal oxygen dependent degradation domain). Reaction mixtures were incubated for 20 h at 37 °C, PHD2 was precipitated by incubation in boiling water for 30 s before NMR analyses. All solutions were buffered with 50 mM Tris-d11(pH 7.5) and 0.02% NaN3in 90% H2O and 10% D2O. Error bars represent s.d. of the mean of triplicate assays. (d) Scheme for 2HG conversion to 2OG. SA, succinic acid; SSA, succinic semialdehyde. Figure 4: Non-enzymatic conversion of ( S )- and ( R )-2HG to 2OG. ( a ) 1 H NMR spectra showing conversion of ( S )-2HG (2-hydroxyglutarate) to 2OG (2-oxoglutarate). The 1 H spectra show the 2OG C H 2 COCO 2 H resonance. Conditions (from top to bottom): 50 μM Fe(II) and 10 mM L -ascorbate; 5 mM ( S )-2HG and 50 μM Fe(II); 5 mM ( S )-2HG and 10 mM L -ascorbate; 5 mM ( S )-2HG; 5 mM ( S )-2HG, 50 μM Fe(II) and 10 mM L -ascorbate. Reaction mixtures were incubated for 20 h at 25 °C. All solutions were buffered with 50 mM Tris -d11 (pH 7.5) and 0.02% NaN 3 in 90% H 2 O and 10% D 2 O. ( b ) Time course of non-enzymatic 2OG production as analysed by 1 H NMR. Conditions: 5 mM ( S )-2HG, 5 μM Fe(II), 2 mM L -ascorbate. ( c ) Succinate and 2OG production (total concentration) in the assay mixtures containing ( R )-2HG. Conditions: 5 mM ( R )-2HG, 5 μM Fe(II), 2 mM L -ascorbate, 4 μM PHD2 (prolyl hydroxylase domain 2), 128 μM CODD ( C -terminal oxygen dependent degradation domain). Reaction mixtures were incubated for 20 h at 37 °C, PHD2 was precipitated by incubation in boiling water for 30 s before NMR analyses. All solutions were buffered with 50 mM Tris -d11 (pH 7.5) and 0.02% NaN 3 in 90% H 2 O and 10% D 2 O. Error bars represent s.d. of the mean of triplicate assays. ( d ) Scheme for 2HG conversion to 2OG. SA, succinic acid; SSA, succinic semialdehyde. Full size image H 2 O 2 and iron promote non-enzymatic 2HG oxidation In addition to 2OG, the NMR assays revealed formation of succinate and another oxidation product, which on the basis of NMR and MS studies was assigned as succinic semialdehyde (SSA) by comparison with a synthetic standard ( Fig. 4d , Supplementary Figs 10 and 11 ) and LC-MS assays ( Supplementary Fig. 12 ). Fenton type chemistry is viable for α-hydroxyacid oxidation [37] ; therefore, the possibility of H 2 O 2 -mediated 2HG oxidation was studied. It was found that 2HG oxidation is enabled by H 2 O 2 to give 2OG, SSA and succinate, and that Fe(II) or Fe(III) are required for this transformation ( Fig. 5 , Supplementary Fig. 13 ). Interestingly, while 2HG oxidation is relatively slow under the conditions of the Fe(II)/ L -ascorbate system (16–20 h or more), the H 2 O 2 -driven reaction is substantially faster (2OG formation was apparent by NMR after 1 h of incubation) ( Supplementary Fig. 14 ). The observed ratio between 2OG and SSA was found to be dependent on the amount of H 2 O 2 added ( Supplementary Figs 15 and 16 ). To investigate whether SSA is the product of further oxidation of 2OG, 2OG oxidation under Fe(II)/ L -ascorbate and Fe(II)/H 2 O 2 conditions was also studied. 2OG was found to be oxidized to succinate, but not to detectable levels of SSA ( Supplementary Figs 17 and 18 ), indicating that SSA formation occurs via an alternative 2HG oxidative pathway. Detectable SSA oxidation to succinate was not observed under these conditions ( Supplementary Fig. 14 ). Therefore the 2HG oxidation reaction most likely proceeds via iron-complex formation. Overall, the results reveal that 2HG is oxidized to 2OG and SSA via (at least) two alternative oxidative pathways, and the ratio of the products depends on the amount of H 2 O 2 present. 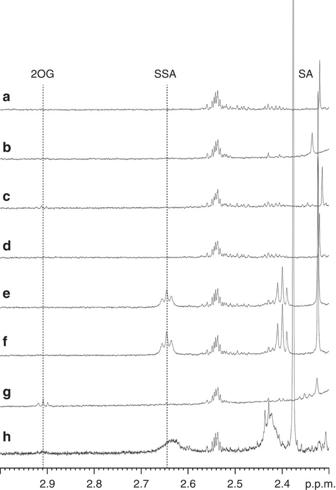Figure 5:1H NMR studies of (R)-2HG oxidation mediated by H2O2. Reaction of (R)-2HG with H2O2in a 90% water 10% D2O mixture ((a) 5 mM (R)-2HG, (b) 5 mM (R)-2HG, 50 μM Fe(II); (c) 5 mM (R)-2HG, 10 mML-ascorbate; (d) 5 mM (R)-2HG, 5 mM H2O2, (e) 5 mM (R)-2HG, 50 μM Fe(II), 5 mM H2O2; (f) 5 mM (R)-2HG, 10 mML-ascorbate, 5 mM H2O2; (g) 5 mM (R)-2HG, 50 μM Fe(II), 10 mML-ascorbate; (h) 5 mM (R)-2HG, 50 μM Fe(II), 10 mML-ascorbate, 5 mM H2O2). 2HG, 2-hydroxyglutarate; 2OG, 2-oxoglutarate; SA, succinic acid; SSA, succinic semialdehyde. Addition of both Fe(II)/L-ascorbate/H2O2leads to impaired 2OG and SSA formation, likely due to competition between different oxidative pathways and/or further oxidation of 2OG and SSA. Figure 5: 1 H NMR studies of ( R )-2HG oxidation mediated by H 2 O 2 . Reaction of ( R )-2HG with H 2 O 2 in a 90% water 10% D 2 O mixture (( a ) 5 mM ( R )-2HG, ( b ) 5 mM ( R )-2HG, 50 μM Fe(II); ( c ) 5 mM ( R )-2HG, 10 mM L -ascorbate; ( d ) 5 mM ( R )-2HG, 5 mM H 2 O 2 , ( e ) 5 mM ( R )-2HG, 50 μM Fe(II), 5 mM H 2 O 2 ; ( f ) 5 mM ( R )-2HG, 10 mM L -ascorbate, 5 mM H 2 O 2 ; ( g ) 5 mM ( R )-2HG, 50 μM Fe(II), 10 mM L -ascorbate; ( h ) 5 mM ( R )-2HG, 50 μM Fe(II), 10 mM L -ascorbate, 5 mM H 2 O 2 ). 2HG, 2-hydroxyglutarate; 2OG, 2-oxoglutarate; SA, succinic acid; SSA, succinic semialdehyde. Addition of both Fe(II)/ L -ascorbate/H 2 O 2 leads to impaired 2OG and SSA formation, likely due to competition between different oxidative pathways and/or further oxidation of 2OG and SSA. Full size image To investigate the role of iron in the observed peroxide driven reaction, we performed stopped-flow UV–vis spectroscopy studies. Transient species absorbing at 240–340 nm, which likely represent different iron oxidation states [38] , were observed during the H 2 O 2 -mediated 2HG oxidation (where the Fe(II)/( R )-2HG mixture was rapidly mixed with H 2 O 2 , Supplementary Figs 19 and 20 ). The formation and degradation of these species occurred over 5 min with the maximum time of their accumulation dependent on the H 2 O 2 concentration, consistent with the NMR 2HG oxidation time course studies ( Supplementary Fig. 14 ), which supports the proposal of iron-mediated conversion of 2HG to 2OG. 2HG-enabled promotion of catalysis by other 2OG oxygenases 2OG oxygenases can produce ROS as a result of incomplete catalytic cycles, which we envisaged could stimulate the observed H 2 O 2 -dependent 2HG oxidation [27] . To investigate this possibility, we studied formation of succinate and 2OG (from 2HG) in the presence of PHD2, with and without CODD substrate ( Fig. 4c ). The total combined concentrations of 2OG and succinate were not increased in the presence of PHD2, suggesting against 2HG oxidation due to ROS production from the PHD2 active site. Owing to consumption of 2OG (produced from 2HG) in the enzymatic reaction, levels of succinate were higher in the presence of PHD2 supporting the proposal that the non-enzymatic oxidation of 2HG occurs at a level sufficient to support PHD2 catalysis. Given the reported ability of ( R )-2HG to activate the PHDs but not other 2OG oxygenases [21] , we investigated whether the observed L -ascorbate-dependent 2HG to 2OG conversion is sufficient to support catalysis by oxygenases other than PHD2. We carried out activity assays with 2HG and L -ascorbate for other human 2OG oxygenases including BBOX1 (γ-butyrobetaine oxygenase, which catalyses the final step in L -carnitine biosynthesis), FIH and the catalytic domain of KDM4A (JMJD2A), an N ε -methyl lysine demethylase. NMR studies on BBOX1 showed that in the absence of 2OG, 2HG addition enables carnitine formation from γ-butyrobetaine (GBB) ( Fig. 6 ). The observed carnitine levels were higher in the case of ( R )-2HG, which is consistent with its lower inhibition potency compared with ( S )-2HG for BBOX1 (IC 50 values are 13.2 mM and 142 μM, for ( R )-2HG and ( S )-2HG, respectively) [14] . Consistent with the fluorescence-based assays on PHD2, addition of BBOX1 to a 2HG/Fe(II)/ L -ascorbate mixture, reacted prior to the enzyme-incubation at 37 °C for 20 h, leads to higher levels of carnitine formation ( Fig. 6 ). As for PHD2 this observation implies that the conversion of 2HG to 2OG is non-enzymatic, with 2OG being formed under the assay conditions. The assays with FIH and KDM4A did not reveal any 2HG-enabled enzyme catalysis at the same concentrations of 2HG/Fe(II)/ L -ascorbate (for which activity was observed for PHD2 and BBOX1), as determined by MS assays. These observations can be rationalized by the 2HG-mediated inhibition of FIH and KDM4A catalysis, and/or by the increased sensitivity of FIH (relative to PHD2) to ROS, including H 2 O 2 , as reported [14] , [21] , [39] . 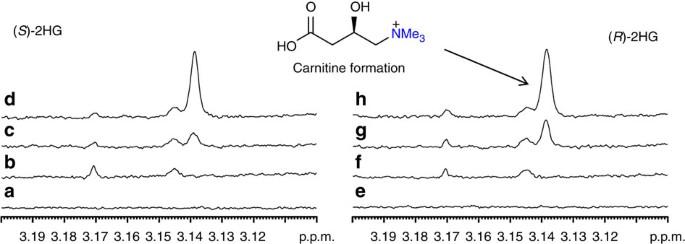Figure 6: Carnitine formation catalysed by BBOX1 in the presence of 2HG. (a) Standards of (S)-2HG (2-hydroxyglutarate) and (e) (R)-2HG; (b) (S)-2HG or (f) (R)-2HG incubated with the assay mixture for 24 h prior to analysis; (c) (S)-2HG or (g) (R)-2HG incubated in the assay mixture with BBOX1 for 24 h prior to analysis; (d) (S)-2HG or (h) (R)-2HG incubated in the assay mixture for 24 h, then treated with BBOX1 and Fe(II) (1:1) and incubated for a further 2 h prior to analysis. The standard assay mixture contained 100 μM GBB (γ-butyrobetaine), 4 mML-ascorbate, 50 μM Fe(II), 80 mM KCl in 50 mM Tris-d11pH 7.5 containing 10% D2O. BBOX1 concentration was 100 nM. (S)-2HG and (R)-2HG were used at a final concentration of 5 mM. Figure 6: Carnitine formation catalysed by BBOX1 in the presence of 2HG. ( a ) Standards of ( S )-2HG (2-hydroxyglutarate) and ( e ) ( R )-2HG; ( b ) ( S )-2HG or ( f ) ( R )-2HG incubated with the assay mixture for 24 h prior to analysis; ( c ) ( S )-2HG or ( g ) ( R )-2HG incubated in the assay mixture with BBOX1 for 24 h prior to analysis; ( d ) ( S )-2HG or ( h ) ( R )-2HG incubated in the assay mixture for 24 h, then treated with BBOX1 and Fe(II) (1:1) and incubated for a further 2 h prior to analysis. The standard assay mixture contained 100 μM GBB (γ-butyrobetaine), 4 mM L -ascorbate, 50 μM Fe(II), 80 mM KCl in 50 mM Tris- d11 pH 7.5 containing 10% D 2 O. BBOX1 concentration was 100 nM. ( S )-2HG and ( R )-2HG were used at a final concentration of 5 mM. Full size image As SSA was observed as a co-product of 2HG oxidation, we studied its influence on 2OG-dependent oxygenases such as PHD2, FIH, KDM4A and BBOX1 (to the extent of our knowledge no data on SSA inhibition of 2OG oxygenases have been reported). SSA caused weak inhibition of all these enzymes (IC 50 values are 4.5 mM, 2.9 mM, 2.8 mM and 267 μM for FIH, PHD2, KDM4A and BBOX1, respectively ( Supplementary Fig. 21 )). Overall, our results clearly demonstrate that the non-enzymatic conversion of 2HG to 2OG can occur. The reaction is promoted by the combination of Fe(II)/Fe(III) and biologically relevant reducing agents such as L -ascorbate and GSH as well as by H 2 O 2 . The 2OG levels produced by non-enzymatic oxidation under our standard steady-state assay conditions are sufficient to support in vitro catalysis by some 2OG oxygenases (PHD2 and BBOX1), but not others (FIH and KDM4A). Although it is not possible to isolate and characterize these reactions within cells, the non-enzymatic conversion of 2HG to 2OG can occur in vitro with physiologically relevant concentrations of Fe(II/III)/reducing agents. We propose that the conditions used by Koivunen et al. [21] likely resulted in non-enzymatic 2HG conversion to 2OG, and that contamination of 2HG with 2OG in commercial samples could also contribute to the 2HG-mediated CODD hydroxylation observed previously and in this study ( Supplementary Fig. 1c ). Although we cannot rule out that it occurs at levels below our limits of detection, we have accrued no evidence for direct 2OG oxygenase catalysed 2HG oxidation; indeed, biophysical studies imply that 2HG binds very weakly to PHD2. In addition, non-enzymatic oxidation should occur without discrimination between enantiomers, which is in accord with our observations. The apparent preference for PHD2 catalysis to proceed in the presence of ( R )- rather than ( S )-2HG observed by Koivunen et al. can be rationalized by the observation that the ( S ) enantiomer is a better PHD2 inhibitor [14] and/or by contamination of some commercial ( R )-2HG batches by 2OG. Similarly with BBOX1, the increased activity with ( R )-, rather than ( S )-2HG, is consistent with the higher inhibition potency for the ( S )-enantiomer [14] . The lack of observed 2HG catalysis with KDM4A and FIH may be due to the relatively stronger inhibition of the former by both ( R )- and ( S )-2HG, and the sensitivity of FIH to ROS, including H 2 O 2 (refs 14 , 39 ). Thus, even though the conversion of 2HG to 2OG is, at least predominantly, non-enzymatic and not enantioselective, the results of the incubation of 2HG with enzymes can appear enantioselective in a condition-dependent manner. The exact mechanisms (likely more than one) of the non-enzymatic oxidation of 2HG are unclear, but probably proceed via iron-complexed ROS [40] , [41] , [42] . Higher rates of reaction were observed with H 2 O 2 replacing L -ascorbate, suggesting the role of L -ascorbate/GSH is to generate ROS, though the exact mechanisms in operation are likely condition-dependent [40] . Further work can focus on whether the non-enzymatic conversion of 2HG to 2OG is of physiological relevance. Given the complexity of 2HG/2OG/TCA cycle metabolism, it is difficult to distinguish between non-enzyme and enzyme-catalysed reactions in cells ( Fig. 7 ) [1] . However, it is well-established that many proteins undergo non-enzymatic oxidative modifications [43] . As indicated in Fig. 7 , it is possible that non-enzymatic reactions may augment the network of identified enzyme-catalysed reactions related to 2HG. The concentrations of the reducing agents at which we observed significant conversion in vitro are probably above those for individual reducing agents in cells [30] . However, taking into account the total cellular concentration of reducing agents capable to promote 2HG oxidation we cannot exclude the possibility of them being sufficient to promote the reaction. Although our in vitro observations indicate that supra-physiological levels of free Fe(II)/Fe(III) (>5 μM) [36] are required for significant levels of 2OG to be formed from 2HG, it is possible that 2HG oxidation may be mediated by complexed iron. Given that non-enzymatic 2HG oxidation is promoted by H 2 O 2 and likely some other ROS, this reaction may be relatively more important under conditions of oxidative stress, mediated by elevated ROS, such as that occurring in hypoxia [44] , [45] , [46] , [47] or in environments of high H 2 O 2 concentration, for example, as occurring in peroxisomes. 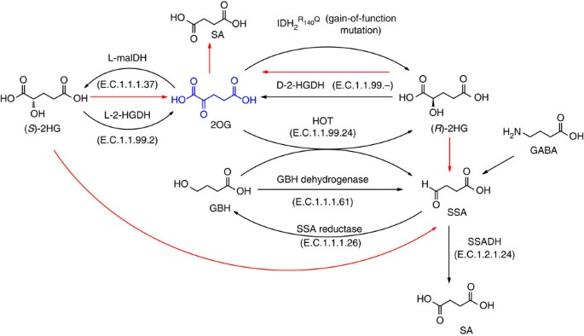Figure 7: Metabolic pathways of (R)- and (S)-2HG. Red arrows represent non-enzymatic transformations observed in this study, black arrows represent identified metabolic pathways.1L-maIDH,L-malate dehydrogenase;L-2-HGDH,L-2-hydroxyglutarate dehydrogenase; IDH2, isocitrate dehydrogenase 2;D-2HGDH,D-2-hydroxyglutarate dehydrogenase; HOT, hydroxyacid-oxoacid transhydrogenase enzyme; GBH, γ-hydroxybutyrate; SSA reductase, succinic semialdehyde reductase enzyme; SSADH, succinic semialdehyde dehydrogenase; GABA, γ-aminobutyric acid. Figure 7: Metabolic pathways of ( R )- and ( S )-2HG. Red arrows represent non-enzymatic transformations observed in this study, black arrows represent identified metabolic pathways. [1] L -maIDH, L -malate dehydrogenase; L -2-HGDH, L -2-hydroxyglutarate dehydrogenase; IDH2, isocitrate dehydrogenase 2; D -2HGDH, D -2-hydroxyglutarate dehydrogenase; HOT, hydroxyacid-oxoacid transhydrogenase enzyme; GBH, γ-hydroxybutyrate; SSA reductase, succinic semialdehyde reductase enzyme; SSADH, succinic semialdehyde dehydrogenase; GABA, γ-aminobutyric acid. Full size image Interestingly, recent work indicates reduction of antioxidant concentrations in IDH-mutated mice [12] . It is thus possible that non-enzymatic Fenton-type chemistry including 2HG/2OG and related metabolites may be involved in the regulation of ROS levels. Indeed, although IDH1/2 mutations have been identified in many cancers [5] , the mechanisms by which they relate to tumorigenesis are unclear. Although, the balance of current evidence suggests that direct inhibition of the HIF hydroxylases by ( R )-2HG is probably not physiologically important [12] , [14] , [15] , the inhibition of chromatin-modifying (or other) 2OG oxygenases by ( R )-2HG with pathophysical consequences remains plausible [14] , [15] , [16] , [48] . It is also proposed that ‘gain-of-function’ IDH mutations may result in depletion of antioxidants including L -ascorbate and GSH, together with perturbation of the NADP + /NADPH ratio, leading to physiologically relevant oxidative stresses [5] . The non-enzymatic chemistry identified here may contribute to the development of such stresses. SSA is a metabolite produced by oxidation of γ-aminobutyric acid (GABA) [49] ( Fig. 7 ). A deficiency in SSA dehydrogenase results from genetic disorders leading to accumulation of SSA in cells where it cannot be further oxidized to succinic acid and subsequently utilized in the TCA cycle [50] . The observation that SSA and succinic acid can be concomitantly produced with 2OG by 2HG oxidation is of interest. The reactive nature of SSA suggests that a potential role for it in cancer metabolism merits investigation. Given that we found that the ratio of 2OG to SSA observed was condition-dependent, it will also be of interest to investigate whether SSA can be detected or its levels vary in cells under conditions of redox stress such as in tumour cells or in highly oxidizing environments such as peroxisomes. It is also notable that in some cases the inhibition potency of SSA for the studied enzymes was higher than for ( R )-2HG, raising the possibility that it might inhibit enzymes in cells. Our results have consequence for the interpretation of the important cellular observations of Koivunen et al. [21] Both HIF-1α and HIF-2α levels were reported to be lower in mid-passage astrocyte cells, in which mutant IDH1 R132H protein was present, compared with wild-type cells. Our results imply that this is unlikely to be due to direct use of ( R )-2HG as a PHD2 co-substrate. Although it does not rationalize the reported resistance of the IDH1 mutant cells to the NOG ( N -oxalyl glycine) precursor DMOG (dimethyloxalyl glycine) [21] , it is possible that the observed effects on HIF-α levels in the astrocyte cells were in part a manifestation of the effect of increased 2HG levels on chromatin-modifying enzymes, including the JmjC demethylases and TET enzymes. The proposal that some of the observed effects on the IDH1 mutant on HIF-α might be mediated via ‘epigenetic processes’ may relate to the observation that HIF-α levels were reported to normalize in later passages (more than passage 20) despite continued production of the mutant IDH1 enzyme and ( R )-2HG. We hope that our results will stimulate further work on the cellular mechanism by which 2HG stimulates PHD activity. Materials ( R )- and ( S )-2-hydroxyglutaric acid disodium salts were from Sigma-Aldrich, UK. The HIF-1α(556–574) CODD peptide, where Met residues in the initial HIF-1α sequence were replaced with Ala, (DLDLEALAPYIPADDDFQL) and HIF-1α(788–822) CAD peptide (DESGLPQLTSYDCEVNAPIQGSRNLLQGEELLRAL) were from GL Biochem (Shanghai) Ltd, China. H3K9me3 (ARK(me3)STGGK) was synthesized as described [51] . Recombinant constructs of catalytic domain of KDM4A (residues 1–359), PHD2 (residues 181–426) and full-length FIH were produced as N -terminally His 6 -tagged protein in Escherichia coli BL21(DE3) cells and purified by Ni-affinity, size-exclusion and cation exchange chromatography as described [52] , [53] , [54] . BBOX1 was expressed and purified as described by Leung et al. [55] Enzymatic assays PHD2, FIH and KDM4A assays were performed at 37 °C as reported [14] . The substrate for PHD2 was the HIF-1α(556–574) CODD 19-mer peptide fragment, wherein the Met residues of the human HIF-1α sequence were substituted for Ala residues to avoid non specific Met oxidation to give a sulfoxide (+16 Da). The substrate for FIH was the HIF-1α(788–822) CAD 35-mer peptide fragment. The substrate for KDM4A was the H3K9me3 peptide. The conditions are described in the Supplementary Table 3 . Samples were analysed using a Waters Micromass MALDI micro MX mass spectrometer (Micromass UK Ltd., Manchester, UK) in reflectron mode with flight tube voltage at 12 kV and reflectron voltage at 5.2 kV. Data were analysed using MassLynx version 4.1. BBOX1 activity assays were performed by NMR. Unless otherwise stated the standard assay mixture contained 100 nM BBOX1, 100 μM GBB (γ-butyrobetaine), 4 mM L -ascorbate, 50 μM (NH 4 ) 2 Fe(SO 4 ) 2 and 80 mM KCl in 50 mM Tris- d11 (pH 7.5) containing 10% D 2 O. SSA inhibition studies were performed by MALDI-TOF-MS and NMR (human BBOX1) using the described conditions [14] . Inhibition of human BBOX1 by SSA was measured by observing carnitine formation by 1 H NMR (Bruker Avance 700). Control reaction mixtures contained 40 μM 2-oxoglutarate disodium salt, 40 μM γ-butyrobetaine hydrochloride, 40 μM ammonium (NH 4 ) 2 Fe(SO 4 ) 2 , 500 μM L -ascorbate, 40 mM KCl and 10% D 2 O in 50 mM pH 7.5 Tris- d11 . Reactions were initiated by addition of human BBOX1 (final concentration 100 nM), the first 1 H NMR spectrum was acquired after 10 min. LC-MS experiments For LC-MS assays, reaction mixtures typically contained 5 mM ( R )- or ( S )-2HG, 50 μM (NH 4 ) 2 Fe(SO 4 ) 2 and variable concentrations (0–10 mM) L -ascorbate/GSH prepared in 50 mM Hepes (pH 7.5), and were incubated for 20 h (37 °C). 2OG production was subsequently measured. Chromatographic separation was performed at 50 °C using a Waters ACQUITY BEH Amide 1.7 μm 2.1 × 100 mm column and a Waters ACQUITYTM ultra-performance liquid chromatography system (Waters Corp., Milford, MA, USA). The following eluents were used: mobile phase A: 10% H 2 O, 90% acetonitrile ( v / v ), 10 mM ammonium formate; mobile phase B: 50% H 2 O, 50% acetonitrile ( v / v ), 10 mM ammonium formate. The elution gradient was 0–10.0 min linear from 10–30% B, and 10.0–12.0 min at 10% B for re-equilibration of the column. A constant flow rate of 0.4 ml min −1 was used. This was directly coupled to a Waters Quattro micro (Micromass UK Ltd) triple quadrupole mass spectrometer in negative ionization mode. The desolvation temperature was set to 250 °C and the source temperature to 120 °C. NMR experiments NMR experiments were conducted at 298 K using a Bruker Avance III 700 MHz spectrometer equipped with a 5 mm inverse TCI cryoprobe and 3 mm diameter MATCH NMR tubes (Bruker). Water suppression was achieved by the excitation sculpting method using a 2 ms 180 degree selective Sinc1.1000 pulse at the H 2 O frequency. Typical experimental parameters were as follows: number of transients 256, relaxation delay 2 s. Unless otherwise stated all samples were 400 μl final volume, consisting of 90% H 2 O and 10% D 2 O with the following concentrations in the reaction mixture: 5 mM 2HG, 50 μM (NH 4 ) 2 Fe(SO 4 ) 2 and 10 mM L -ascorbate. The non-enzymatic reaction was started by addition of hydrogen peroxide with 5 mM as standard final concentration and then monitored for 2 h by 1 H NMR at 298 K. The CPMG (Carr–Purcell–Meiboom–Gill) displacement experiments were conducted using the AV700 instrument and 3 mm MATCH NMR tubes [32] . The PROJECT-CPMG sequence (90° x –[ τ –180° y – τ –90° y – τ –180° y – τ ] n –acq) was applied as described by Aguilar et al. [56] Typical experimental parameters were as follows: total echo time 48 ms ( τ =2 ms, n =6), acquisition time 2.94 s, relaxation delay 2 s and number of transients 128. Water suppression was achieved by presaturation. UV–vis spectroscopy experiments Absorption spectra were acquired using a Cary Varian 4000 UV–vis spectrophotometer at 22 °C with 0.1 mM PHD2, 0.1 mM Fe(II) and 0.5 mM 2OG or ( R )/( S )-2HG in deoxygenated 50 mM Hepes (pH 7.5). The buffer and enzyme were deoxygenated according to the described procedure [22] . All other solutions were prepared in an anaerobic glove box (Belle Ltd., UK). Non-denaturing ESI-MS experiments Non-denaturing ESI-MS experiments were performed as described [57] . PHD2 was buffer-exchanged into 15 mM ammonium acetate (pH 7.5). Data were analysed using MassLynx 4.0. Amino acid analysis Amino acid analysis was performed as previously described [58] . An extracted ion chromatogram was created using m / z value corresponding to AQC-derivatized hydroxyproline (304±0.2 Da). Three chromatograms were acquired for every sample. The limit of detection for the method was determined to be ~1 pmol μl −1 . Stopped-flow UV–vis spectroscopy experiments Solutions of 10 mM ( R )-2HG, 0.2 mM Fe(II) were prepared in Milli-Q water and rapidly mixed with 2 mM H 2 O 2 at 1:1 ratio in a stopped-flow apparatus (Applied Photophysics, Leatherhead, UK). Subsequent analysis used an SX20 stopped-flow spectrometer and spectra were recorded over time up to 500 s using a photodiode array detector. All assays were performed at least in triplicate. Synthesis of SSA SSA was prepared from methyl 4,4-dimethoxybutyrate (Sigma-Aldrich). The starting material (100 mg) was dissolved in 5 ml of tetrahydrofurane and treated with 3 ml of 1 M lithium hydroxide. The reaction mixture was stirred overnight and then tetrahydrofurane was removed in vacuo . The water phase was acidified with concentrated HCl and stirred for a further 6 h. The solution was concentrated to 1 ml in vacuo and purified on HPLC (reverse phase column, gradient 10% of B in 15 min where A: 0.05% TFA in H 2 O, B: 0.1% TFA in acetonitrile, retention time 9 min). Fractions containing the product were freeze-dried to yield SSA as an off-white oil. 1 H NMR (500 MHz, D 2 O ) δ p.p.m. 5.00 (t, J =5.5), 2.40 (t, J =7.5), 1.82 (dt, J 1 =7.5, J 2 =5.5); 13 C NMR (125 MHz, D 2 O ) δ p.p.m. 177.5, 89.1, 31.9, 28.8. LC-MS analysis retention time is 1.15 min (Waters ACQUITY BEH Amide 1.7 μm 2.1 × 100 mm column, mobile phase A: 10% H 2 O, 90% acetonitrile ( v / v ), 10 mM ammonium formate; mobile phase B: 50% H 2 O, 50% acetonitrile ( v / v ), 10 mM ammonium formate), mass—101.2 (negative ion mode). How to cite this article: Tarhonskaya, H. et al. Non-enzymatic chemistry enables 2-hydroxyglutarate-mediated activation of 2-oxoglutarate oxygenases. Nat. Commun. 5:3423 doi: 10.1038/ncomms4423 (2014).